Dust inputs and bacteria influence dissolved organic matter in clear alpine lakes Remote lakes are usually unaffected by direct human influence, yet they receive inputs of atmospheric pollutants, dust, and other aerosols, both inorganic and organic. In remote, alpine lakes, these atmospheric inputs may influence the pool of dissolved organic matter, a critical constituent for the biogeochemical functioning of aquatic ecosystems. Here, to assess this influence, we evaluate factors related to aerosol deposition, climate, catchment properties, and microbial constituents in a global dataset of 86 alpine and polar lakes. We show significant latitudinal trends in dissolved organic matter quantity and quality, and uncover new evidence that this geographic pattern is influenced by dust deposition, flux of incident ultraviolet radiation, and bacterial processing. Our results suggest that changes in land use and climate that result in increasing dust flux, ultraviolet radiation, and air temperature may act to shift the optical quality of dissolved organic matter in clear, alpine lakes. Remote lakes have been recognized as sensors of global change [1] , [2] , [3] and are key freshwater reference sites for global-scale processes, owing to their location outside of direct human influence. However, remote lakes are also subject to the deposition of atmospheric pollutants, mineral dust, and organic matter transported by aeolian processes [4] , [5] , [6] , [7] . Despite the relatively small area covered by lakes and other freshwater ecosystems on a global basis, the movement of carbon through these ecosystems is dynamic and relevant for regional and global carbon budgets [8] . Dissolved organic matter (DOM), the major form of aquatic organic carbon, has key functions in aquatic ecosystems that include supplying energy to support the aquatic food web and absorbing ultraviolet radiation and light, thereby regulating their penetration in the water column. DOM in lakes located below treeline is strongly influenced by catchment vegetation inputs [9] . In contrast, alpine lakes (that is, above treeline) are often located above the atmospheric boundary layer (1,000 to 1,500 m a.s.l. ), and generally on barren catchments or catchments with poorly developed soils and vegetation. Therefore, autochthonous DOM production, atmospheric inputs of organic matter, and climatic controls may have a greater bearing on dissolved organic carbon (DOC) concentration and quality in alpine lakes than inputs from terrestrial vegetation. In this respect, our understanding of atmospheric influences on DOM dynamics in alpine lakes is limited. Thus far, it has been recognized that organic matter travelling in Saharan dust plumes represents an important input of DOM to alpine lakes, such as those in the Sierra Nevada, Spain [10] . Estimates of the organic fraction associated with dust events vary widely, but long-term monitoring studies of atmospheric deposition close to dust sources agree that at least 8% to 14% [11] , [12] , of the particulate matter is organic carbon. The organic fraction is mainly attributed to anthropogenic pollutants partitioning onto the mineral surface, which can occur in fine (<10 μm in diameter) [14] or coarse (>10 μm in diameter) [11] , [13] particles. This organic fraction has also been associated with crustal source areas, such as soils [7] , [11] , and may originate from erodible lake sediments [15] and primary biological aerosols, such as bacteria, fungi and pollen [16] , much of which is larger than 10 μm. In addition to potentially increasing dust transport [17] and associated atmospheric deposition of nutrients and organic matter, rising temperatures associated with climate change will reduce ice cover [3] , accelerate glacial melt [18] , increase water residence time [19] , and consequently increase ultraviolet exposure [20] and atmospheric exposure in general. Together, these conditions may alter the chemical and optical properties of DOM (that is, chromophoric DOM or CDOM). Sources and spatiotemporal variability of DOM have been tracked successfully with optical properties obtained from ultraviolet-visible absorbance and fluorescence spectroscopy measurements, such as molar absorption, spectral slopes [21] , [22] , fluorescence indices [23] and fluorescent components found in excitation–emission matrices (EEMs) [24] , [25] . These optical properties also impart valuable biological and chemical information about DOM, such as degree of aromaticity, bioavailability, light attenuation and molecular weight. For example, slopes of the ultraviolet-visible absorption curve provide information about algal and terrestrial humic contributions to the DOM pool [22] and the proportion of low molecular weight compounds that absorb at short wavelengths to high-molecular weight compounds that absorb at longer wavelengths [21] . These and other optical spectroscopic measurements are more sensitive parameters to environmental changes than measurements of DOC concentration alone [21] , [26] . To better understand the dominant controls on DOM and its optical properties in remote aquatic ecosystems, we sampled 86 globally distributed remote lakes and evaluated relationships between DOM and factors that change over latitude, such as the Ozone Monitoring Instrument (OMI) aerosol index (AI) [27] , OMI clear-sky ultraviolet radiation (CS ultraviolet λ ) [28] , mean annual precipitation, and other external factors, such as the percentage of vegetation cover and elevation, but also within-lake factors, such as water residence time, chlorophyll- a (Chl a ) concentration, and bacterial abundance (BA), ( Fig. 1 ; Supplementary Tables S1–S6 ). Our sampling included alpine lakes within the Saharan dustbelt (Atlas, Sierra Nevada, Pyrenees, and Tyrolean Alps) and within other aerosol influences (Patagonia), as well as remote lakes at low elevations (<1,000 m a.s.l.) outside of major dust influences (Antarctica and the Arctic) ( Fig. 1; Supplementary Figure S1 ). This choice of remote lakes in catchments containing little or no vegetation provided a latitudinal transect from both the northern and southern hemispheres that allowed us to explore spatial gradients in DOC concentration and optical properties without an overprinting effect from catchment vegetation. Also, very clear (low DOC) lakes were included in the dataset to increase the probability of detecting influences on DOM optical properties. Here we show that atmospheric dust inputs and ultraviolet radiation combined with bacterial processing of DOM may jointly influence the observed latitudinal trends in the optical properties of alpine lake DOM. 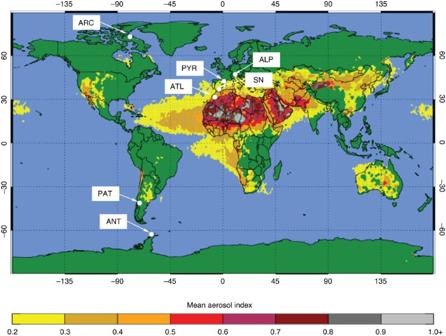Figure 1: Map of study sites and global distribution of aerosols. Approximate location (white dots) of lakes (ATL=Atlas (2 lakes,N=2); SN=Sierra Nevada (25 lakes,N=25); PYR=Pyrenees (16 lakes,N=28); ALP=Tyrolean Alps (17 lakes,N=38); PAT=Patagonian Andes (6 lakes,N=6); ANT=Antarctica (15 lakes,N=15), ARC=Canadian Arctic (6 lakes,N=6)) sampled in this study and contours of the annual mean aerosol index (AI) obtained by the NASA–KNMI Ozone Monitoring Instrument. AI values <0.2 removed for clarity. Monthly and annual mean weighted AI values are shown inSupplementary Tables S1andS2,and calculations are described in theSupplementary Methods.N=number of samples. Figure 1: Map of study sites and global distribution of aerosols. Approximate location (white dots) of lakes (ATL=Atlas (2 lakes, N =2); SN=Sierra Nevada (25 lakes, N =25); PYR=Pyrenees (16 lakes, N =28); ALP=Tyrolean Alps (17 lakes, N =38); PAT=Patagonian Andes (6 lakes, N =6); ANT=Antarctica (15 lakes, N =15), ARC=Canadian Arctic (6 lakes, N =6)) sampled in this study and contours of the annual mean aerosol index (AI) obtained by the NASA–KNMI Ozone Monitoring Instrument. AI values <0.2 removed for clarity. Monthly and annual mean weighted AI values are shown in Supplementary Tables S1 and S2, and calculations are described in the Supplementary Methods . N =number of samples. Full size image Latitudinal trends in DOM optical properties In alpine lakes, we observed significant latitudinal trends for DOC concentration and optical properties of DOM, namely ultraviolet absorption ( a 250 ), total fluorescence ( F total ), spectral slope curve values ( S cλ ) [22] , and the spectral slope ratio ( S R ) [21] ( Fig. 2 Supplementary Tables S7 and S8 ). By contrast, the Arctic and Antarctic lakes we sampled lie outside of the main aerosol influence (AI=0) and did not reflect these latitudinal trends ( Fig. 2 ). Additionally, Arctic lakes were located in the tundra with a greater fraction of their catchments covered with vegetation ( Supplementary Table S3 ). Thus, their higher allochthonous terrestrial C inputs likely also contribute to their higher spectral slope, ultraviolet absorption, and DOC concentration. 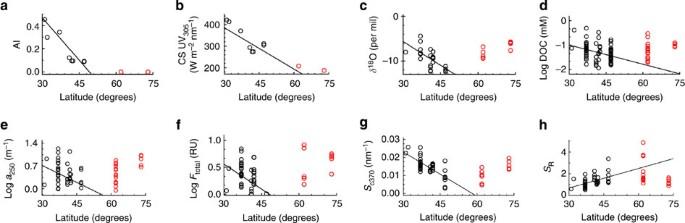Figure 2: Changes in lake characteristics and DOM properties with latitude. Latitudinal gradients of external factors, (a) aerosol index (AI) and (b) clear-sky ultra violet radiation (CS UV305), lake characteristics, (c) stable isotope of oxygen (δ18O), and (d) dissolved organic carbon (log DOC) concentration, and DOM optical properties, (e) absorption (loga250), (f) total fluorescence (logFtotal), (g) spectral slope curve at 370 nm (Sc370), and (h) spectral slope ratio (SR) in alpine (black circles) and polar (red circles) lakes. Regression lines indicate significant relationships between latitude and AI (r=−0.83,P<0.001;N=115), CS UV305(r=−0.61,P<0.001;N=115),δ18O (r=−0.43,P=0.005;N=41), log DOC (r=−0.29,P=0.019;N=65), loga250(r=−0.33,P=0.025;N=46), logFtotal(r=−0.38,P=0.012;N=43),Sc370(r=−0.76,P<0.001;N=49), andSR(r=0.51,P<0.001;N=45).N=number of samples. North and South latitudes are pooled and samples collected at depths >2 m were excluded. Figure 2: Changes in lake characteristics and DOM properties with latitude. Latitudinal gradients of external factors, ( a ) aerosol index (AI) and ( b ) clear-sky ultra violet radiation (CS UV 305 ), lake characteristics, ( c ) stable isotope of oxygen ( δ 18 O), and ( d ) dissolved organic carbon (log DOC) concentration, and DOM optical properties, ( e ) absorption (log a 250 ), ( f ) total fluorescence (log F total ), ( g ) spectral slope curve at 370 nm ( S c370 ), and ( h ) spectral slope ratio ( S R ) in alpine (black circles) and polar (red circles) lakes. Regression lines indicate significant relationships between latitude and AI ( r =−0.83, P <0.001; N =115), CS UV 305 ( r =−0.61, P <0.001; N =115), δ 18 O ( r =−0.43, P =0.005; N =41), log DOC ( r =−0.29, P =0.019; N =65), log a 250 ( r =−0.33, P =0.025; N =46), log F total ( r =−0.38, P =0.012; N =43), S c370 ( r =−0.76, P <0.001; N =49), and S R ( r =0.51, P <0.001; N =45). N =number of samples. North and South latitudes are pooled and samples collected at depths >2 m were excluded. Full size image The spectral slope ratio ( S R ) is a metric from ultraviolet-visible absorption spectroscopy, where the slope in the short-wavelength range ( S 275–295 ), low-molecular weight region is related to the slope in the longer wavelength range ( S 350–400 ), higher molecular weight (>1,000 Daltons) region [21] . The spectral slope curve at 370 nm ( S c370 ) is similar in position to peaks of reference humic and fulvic acids reported in ref. 22 . Excluding polar lakes, the most striking latitudinal changes ( Fig. 2 ) were in the S R , which increased by almost two units from Lac d'Ifni in the Atlas Mountains of Morocco to Gossenköllesee in the Tyrolean Alps, and the spectral slope curve at 370 nm ( S c370 ), which decreased substantially with increasing latitude ( Fig. 2 ; Supplementary Table S8 ). AI and clear-sky ultraviolet radiation were significantly related to S c370 ( r =0.62, P <0.001, N =49 and r =0.53, P <0.001, N =49, respectively) and S R ( r =−0.51, P =0.001, N =45 and r =−0.41, P =0.005, N =45, respectively) and increased significantly with proximity to the Saharan dust source ( Fig. 2 ). Any correlation between the percentage of vegetation cover in the lake catchments and spectral parameters from absorbance was lacking in alpine lakes. This suggests that terrestrially derived DOM from the catchment did not significantly contribute to these changes in spectral slope curve and spectral slope ratio. Fluorescence characteristics Fluorescence characteristics of dry deposition samples were strikingly similar to those of alpine lakes on barren, rocky terrain and quite unlike those of polar lakes. In particular, three-dimensional excitation–emission matrix spectra (EEMs) of water soluble organic carbon (WSOC) from dry deposition and DOM in clear, alpine lake samples had intense peaks in the short excitation and emission wavelength range typically associated with amino-acid fluorescence and less intense peaks at longer emission wavelengths associated with the presence of humic substances ( Fig. 3 ). Parallel factor analysis (PARAFAC) modelling ( Supplementary Figs S1 and S2 ) identified that fluorescence in the short excitation and emission range, mainly due to fluorescent components 3 (tryptophan-like) and 4 (tyrosine-like), represented 54±12% ( N =9; Supplementary Table S9 ) of the total fluorescence of atmospheric WSOC and 50±19% ( N =40) of the total fluorescence of DOM from alpine lakes located on barren, rocky terrain ( Fig. 3 ). In polar lakes, the combined fluorescence of components 3 and 4 represented only 15±10%. Fluorescence spectra of biological and chemical organics that may be found in the atmosphere, such as pollen, airborne bacteria, formaldehyde, hydrogen peroxide, urban aerosols and diesel exhaust, were measured ( Supplementary Fig. S2 ). Of the compounds examined here, the fluorescence in the short excitation and emission range in our alpine lake samples most closely resembled fluorescence from pollen, airborne bacteria, and formaldehyde ( Supplementary Fig. 23 ). 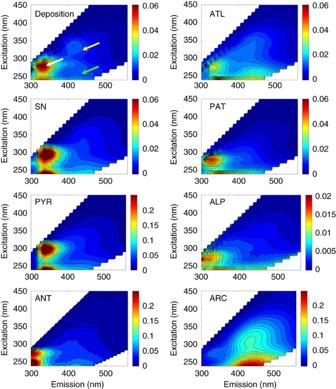Figure 3: Similarities in fluorescence spectra of atmospheric deposition and alpine lake DOM. Representative EEMs of water soluble organic carbon from dry deposition (Deposition) collected at the Sierra Nevada Observatory on 8 July 2008, DOM from lakes on rocky catchments of the Atlas (ATL: Lac D'Ifni), Sierra Nevada (SN: Cuadrada), Patagonia (PAT: Tempanos), the Pyrenees (PYR: Ibonet Perramó), and the Alps (ALP: Faselfad 4) show well-resolved fluorescence peaks at short excitation and emission wavelengths. For comparison, DOM from low-elevation lakes on partially vegetated catchments in Antarctica (ANT: Somero) and the Arctic (ARC: Bylot 40) are shown. Arrows point to low excitation/emission (amino-acid-like) (white), humic-acid-like (yellow), and fulvic-acid-like (green) peaks according to ref.24. Figure 3: Similarities in fluorescence spectra of atmospheric deposition and alpine lake DOM. Representative EEMs of water soluble organic carbon from dry deposition (Deposition) collected at the Sierra Nevada Observatory on 8 July 2008, DOM from lakes on rocky catchments of the Atlas (ATL: Lac D'Ifni), Sierra Nevada (SN: Cuadrada), Patagonia (PAT: Tempanos), the Pyrenees (PYR: Ibonet Perramó), and the Alps (ALP: Faselfad 4) show well-resolved fluorescence peaks at short excitation and emission wavelengths. For comparison, DOM from low-elevation lakes on partially vegetated catchments in Antarctica (ANT: Somero) and the Arctic (ARC: Bylot 40) are shown. Arrows point to low excitation/emission (amino-acid-like) (white), humic-acid-like (yellow), and fulvic-acid-like (green) peaks according to ref. 24 . Full size image The role of bacteria Concomitant with aerosol and climatic controls, lake bacteria also affect DOM properties. BA increased with elevation in alpine lakes ( Fig. 4a ) and also increased with proximity to the Saharan dust source. Log BA was higher in lakes with longer water residence time (using δ 18 O values as a proxy for this parameter; r =0.74, P =0.004, N =13). Further, significant correlations between log BA and log DOC concentration ( Fig. 4b ), log a 250 ( Fig. 4c ), and log F total ( Fig. 4d ) indicate important connections between BA and DOM optical properties in alpine lakes. 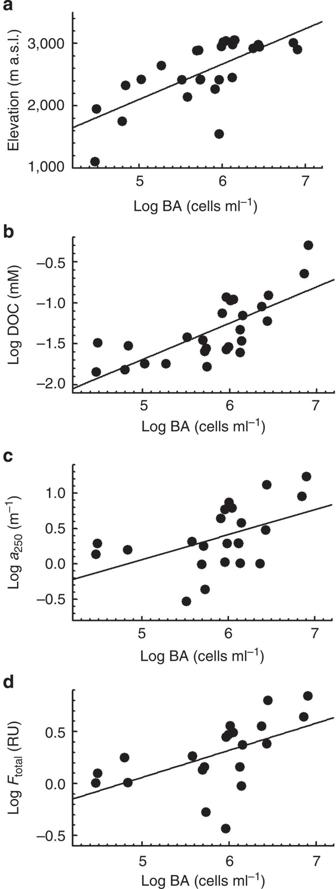Figure 4: Bacterial abundance trends and influence on DOM production. Scatterplots showing significant relationships between bacterial abundance (log BA) and (a) elevation (r=0.72,P<0.001,N=26), (b) DOC concentration (log DOC) (r=0.74,P<0.0001,N=26), (c) absorption (loga250) (r=0.49,P<0.017,N=23), and (d) total fluorescence (logFtotal) (r=0.55,P=0.01,N=21) in alpine lakes.N=number of samples. Samples collected at depths >2 m were excluded. Figure 4: Bacterial abundance trends and influence on DOM production. Scatterplots showing significant relationships between bacterial abundance (log BA) and ( a ) elevation ( r =0.72, P <0.001, N =26), ( b ) DOC concentration (log DOC) ( r =0.74, P <0.0001, N =26), ( c ) absorption (log a 250 ) ( r =0.49, P <0.017, N =23), and ( d ) total fluorescence (log F total ) ( r =0.55, P =0.01, N =21) in alpine lakes. N =number of samples. Samples collected at depths >2 m were excluded. Full size image The latitudinal pattern in DOM optical properties observed in alpine lakes appears to be a function primarily of atmospheric dust deposition and secondarily of the flux of incident ultraviolet radiation (multiple regression analyses in Supplementary Tables S10–S12 ). These external factors may exert controls on DOM quantity and quality in high-elevation lakes in several non-exclusive ways. First, we hypothesize that dust deposition, which is highest near dust sources [29] , may directly supply high-molecular weight CDOM to remote lakes, and that the changes observed in DOM optical properties with decreasing latitude result from proximity to global dust sources, most notably the Sahara and Sahel. Indeed, long-term monitoring studies show that dust deposition and coarse particulate matter aerosols originating in North Africa comprise on average >10% organic carbon [11] , [12] , and represent a major fraction of the DOM input to a clear, alpine lake within the Saharan dustbelt [4] . This atmospheric influence on the DOM quality of alpine lakes is supported by the significant positive relationships between AI and S c370 and S R and the significant increase in S c370 and decrease in S R with proximity to the Saharan dust source ( Fig. 2 ). Taken together with the association of high S c370 and low S R with higher molecular weight, humic DOM [21] , [22] , these spatial trends indicate greater input, production, or selective preservation of high-molecular weight, humic-like substances with proximity to the Sahara. Moreover, the low S R values in alpine lakes located closer to the Sahara are consistent with low S R values (mean of 1.86±0.97, N =6; Supplementary Table S9 ) in WSOC from dry deposition collected within the Saharan dustbelt. Three-dimensional fluorescence spectra of WSOC from dry deposition were similar to those of DOM in clear, alpine lake samples and unlike those of polar lakes ( Fig. 3 ). EEMs of WSOC and DOM in alpine lakes contained peaks in the short excitation and emission wavelength range, which resemble those of bioaerosols, such as bacteria and pollen, and oxidized organic compounds in the atmosphere ( Supplementary Fig. S2 ), and at longer emission wavelengths associated with the presence of humic substances ( Fig. 3 ). Therefore, dust transport may be a vector for organic constituents from multiple sources that may either be mobilized at the dust source or partition to the mineral surface during transport [11] . Second, the correlations between clear-sky ultraviolet radiation and optical properties of alpine lake DOM may reflect the increasing importance of photochemical processes with decreasing latitude. The increase in S c370 values and other S cλ values between 350 and 400 nm, representative of high-molecular weight compounds [21] and humic substances [22] , with increasing ultraviolet radiation is consistent with results from CDOM photochemical experiments [22] , and may, more specifically, indicate photohumification processes. In clear marine waters, photohumification or the oxidation, condensation, and transformation of dissolved triglycerides and fatty acid compounds into humic substances by ultraviolet radiation has been documented [30] . In the clear alpine lakes of this study, S c370 also increased with greater δ 18 O values ( r =0.57, P =0.005, N =21), which may further reflect greater exposure to both ultraviolet radiation and atmospheric deposition with longer water residence. In addition to signalling longer water residence time, the increasing δ 18 O values with decreasing latitude ( Fig. 2 ) may be indicative of shorter periods of ice cover, which imply longer atmospheric exposure in those lakes closer to both the equator and the Saharan dust source. Optical properties of DOM in alpine lakes may also be influenced by the microbial response to dust deposition. Dust deposition supplies alpine lakes with nutrients, particularly phosphorus, that stimulate phytoplankton and bacterial growth [31] , [32] . Phytoplankton exudates of organic substances and their subsequent bacterial processing [32] , as well as the direct release of mycosporine-like amino acids [33] , [34] under ultraviolet stress are known to be linked to CDOM and fluorescent DOM ( Supplementary Fig. S3 ) production. Perhaps of equal importance for alpine lakes is the potential stimulation of bacterial growth by atmospheric deposition of DOM and nutrients. In our study, strong correlations between bacterial abundance, elevation, and δ 18 O suggest that at high elevations, fertilization by dust may be pronounced because of minimal catchment vegetation influences and relatively greater exposure to atmospheric deposition. Further, the significant relationship between log BA and log DOC concentration taken together with the increase in log BA with increasing AI ( r =0.62, P =0.001, N =26) and increasing log DOC concentrations with AI ( r =0.40, P =0.004, N =62) point to DOM from atmospheric deposition as an energy source for bacterial growth. The relationships between BA and absorption at 250 nm and at other wavelengths ( Supplementary Table S7 ) further suggest that bacteria are producing CDOM. Even though BA is not a surrogate for bacterial activity, this parameter may provide a coarse indication of bacterial production in these alpine lakes. Significant positive relationships between BA and F total for alpine lakes extend this notion to bacterial production of fluorescent DOM. Alpine and other remote lakes have been used as reference sites and recent studies have emphasized their importance as sensors of global change [1] , [3] . There is increasing evidence that these “pristine” lakes are vulnerable to climatic and atmospheric influences. More than a decade ago, it was hypothesized that changes in dust deposition and climate warming will be key factors for the development of alpine lakes [35] . Now, we observe that dust exerts direct and indirect influences on lake DOM, with water residence time and the duration of ice cover further acting to control exposure of lakes to dust and its associated organic and inorganic constituents. Because the chemical character of DOM influences its bioavailability, its role in light attenuation in the water column, and consequently the water quality of alpine lakes, the observed geographic patterns in DOM and their relation to dust deposition are of great consequence for these remote systems. Beyond the importance that DOM has on lake ecosystems, what we observe is a strong connection between alpine lakes and the atmosphere that may be relevant in terms of detecting changes in the atmospheric cycling of organic carbon, for instance, or in the role of dust as a vector for the transport of nutrients and pollutants at a global scale. Although the polar lakes included in this study did not reflect an atmospheric influence in their DOM optical properties due to their position at low elevations and outside the extent of the dustbelt, these systems are also particularly vulnerable to climatic changes, which are expected to be relatively large at high latitudes [36] . Our new evidence that alpine lake bacteria may be both influenced by the organic carbon in dust deposition and may influence alpine lake optical properties by producing chromophoric organic compounds ultimately has major implications for carbon cycling. The higher bacterial abundance at higher elevations and presumably under more extreme environmental conditions (for example, ultraviolet radiation) is an unexpected result that merits further study, particularly in the context of microbial food-web dynamics in alpine lakes. Rising temperatures in the future are likely to steer remote lake microbial dynamics toward greater productivity [36] , [37] , whereas land use change and other disturbances that exacerbate the mobilization and transport of dust [38] , [39] and its associated organic and inorganic constituents will have additional consequences for alpine lake trophic dynamics. Sample collection and DOM characterization measurements Water samples were collected from alpine and polar lakes ( Supplementary Table S1 ) and filtered with pre-combusted glass fibre filters (GF/F). Atmospheric dry deposition samples were collected using an automatic wet/dry deposition collector located at 2,896 m a.s.l. at the Sierra Nevada Observatory, a site of frequent Saharan dust intrusions. Water-soluble organic carbon was extracted from dry deposition using ultra-pure water and filtered through pre-combusted GF/F filters. DOC concentrations were measured on GF/F filtered, acidified samples with Shimadzu TOC analysers. Ultraviolet-visible absorbance was measured on GF/F filtered, unacidified samples using a Perkin Elmer Lambda 40 and Beckman DU-640 ultraviolet-visible spectrophotometers. The Naperian absorption coefficient and spectral slope ratio were calculated according to ref. 21 and spectral slope curves were calculated as described in ref. 22 with 20 nm offsets ( Supplementary Fig. S4 ). Fluorescence scans used in PARAFAC modelling were measured on GF/F filtered, unacidified samples using a JY Horiba Fluoromax-4 spectrofluorometer with instrument-specific corrections applied during spectral acquisition. Excitation–emission matrices were normalized to the area under the Raman curve, inner filter corrected, and blank subtracted. For PARAFAC modelling [25] ( Supplementary Fig. S5 and Supplementary Table S13 ) and generation of measured, modelled, and residual EEMs ( Supplementary Fig. S6 ), the areas of Rayleigh scatter were excised and outliers were removed from the model. Other parameters Samples were analysed for oxygen isotopic composition using the CO 2 –H 2 O equilibration method. Chlorophyll a concentrations were obtained by measuring absorbance of acetone-extracted GF/F filters or by high-pressure liquid chromatography on methanol-extracted GF/F filters. Bacterial abundance was measured either by flow cytometry or epifluorescence microscopy with DAPI staining. The percentage of vegetation cover in lake catchments was estimated from photographic surveys. The clear-sky ultraviolet radiation and aerosol index data were obtained from observations by the NASA–KNMI (Netherlands Royal Meteorological Institute) Ozone Monitoring Instrument. More detailed methods are provided in the online Supplementary Information . How to cite this article: Mladenov, N. et al . Dust inputs and bacteria influence dissolved organic matter in clear alpine lakes. Nat. Commun. 2:405 doi: 10.1038/ncomms1411 (2011).